SUMO1 modification of PTEN regulates tumorigenesis by controlling its association with the plasma membrane The membrane association of the tumour suppressor phosphatase and tensin homologue (PTEN) is required to oppose the phosphatidylinositol-3-kinase/AKT pathway by dephosphorylation of phosphatidylinositol-3,4,5-triphosphate (PIP3). How cytosolic PTEN interacts with its main substrate, PIP3, localized at the inner face of plasma membrane remains unclear. Here we show that PTEN is covalently modified by SUMO1 at both K 266 and K 254 sites in the C2 domain of PTEN. SUMO1 modification at K 266 located in the CBR3 loop, which has a central role in PTEN membrane association, mainly facilitates cooperative binding of PTEN to the plasma membrane by electrostatic interactions. This results in the downregulation of the phosphatidylinositol-3 kinase/AKT pathway and consequently, suppression of anchorage-independent cell proliferation and tumour growth in vivo . Our data demonstrate a molecular mechanism whereby SUMO1 modification is required for PTEN tumour suppressor function by controlling PTEN membrane association and regulation of the phosphatidylinositol-3 kinase/AKT pathway. The tumour suppressor gene PTEN (phosphatase and tensin homologue deleted on chromosome 10) is one of the most frequently deleted or mutated in diverse human tumours. PTEN is composed of N-terminal phosphatase domain, C2 domain and C-terminal tail domain ( Fig. 1a ). PTEN binding to the plasma membrane is a critical regulatory step for PTEN function in antagonizing the phosphatidylinositol-3 kinase (PI3K) signalling pathway by converting phosphatidylinositol 3,4,5-triphosphate (PIP3) to phosphtidylinositol 4,5-biphosphate (PIP2) [1] , [2] . PTEN is mainly found in the cytosol and nucleus. Several studies have shown that under normal conditions, only a small fraction of cytosolic PTEN is dynamically bound to the plasma membrane, because PTEN in a constrained conformation has a low affinity for membrane binding [2] , [3] . It is still poorly understood how cytosolic PTEN interacts with its main substrate PIP3 localized at the inner face of plasma membrane, although several elements/factors, including the CBR3 loop in the C2 domain [4] , [5] , [6] , N-terminal PIP2-binding motif ( Fig. 1a ) and PIP2 [6] , [7] , C-terminal tail phosphorylations [2] , [3] , [8] , [9] , [10] and integrity of the phosphatase [2] , [3] , have been suggested to be involved in the membrane binding and activation of PTEN. 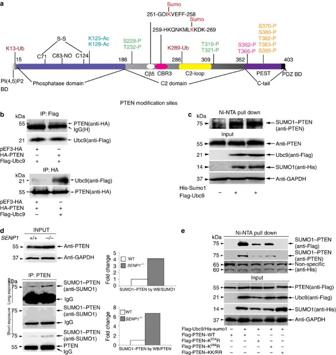Figure 1: PTEN is SUMOylated at K254and K266in vivo. (a) Post-translational modification sites of human PTEN protein. Evolutionarily conserved SUMOylation motif lysines are shown in red. (b) Exogenous PTEN binds to SUMO-conjugating enzyme Ubc9. Lysates from 293T cells transfected with Flag-Ubc9, with or without HA-PTEN were used for immunoprecipitation (IP) with anti-Flag and detected by western blotting. Reciprocally, lysates from 293T cells transfected with HA-PTEN, with or without Flag-Ubc9 were used for IP with anti-HA and detected by western blotting. (c) HeLa cells transfected with or without Flag-Ubc9/His-SUMO1 were lysed and treated with Ni2+-NTA resin for SUMOylation assays11. (d)SENP1+/+andSENP1−/−MEFs were starved for 24 h and lysed. Lysates as an input were immunoblotted with anti-PTEN and anti-GAPDH antibodies. Lysates were also immunopreciptated with PTEN antibody and then immunoblotted with SUMO1 antibody (with short or long exposure). After stripping, the same membrane was detected with PTEN antibody. Quantification was analysed by ImageJ (V1.45) and the SUMO1–PTEN bands were normalized with the IgG bands. (e) 293T cells co-transfected with PTEN–WT or mutants K254R, K266R and K254R/K266R (KK/RR) with or without Flag-Ubc9/His-SUMO1 were lysed and treated for SUMOylation assays. Figure 1: PTEN is SUMOylated at K 254 and K 266 in vivo . ( a ) Post-translational modification sites of human PTEN protein. Evolutionarily conserved SUMOylation motif lysines are shown in red. ( b ) Exogenous PTEN binds to SUMO-conjugating enzyme Ubc9. Lysates from 293T cells transfected with Flag-Ubc9, with or without HA-PTEN were used for immunoprecipitation (IP) with anti-Flag and detected by western blotting. Reciprocally, lysates from 293T cells transfected with HA-PTEN, with or without Flag-Ubc9 were used for IP with anti-HA and detected by western blotting. ( c ) HeLa cells transfected with or without Flag-Ubc9/His-SUMO1 were lysed and treated with Ni 2+ -NTA resin for SUMOylation assays [11] . ( d ) SENP1 +/+ and SENP1 −/− MEFs were starved for 24 h and lysed. Lysates as an input were immunoblotted with anti-PTEN and anti-GAPDH antibodies. Lysates were also immunopreciptated with PTEN antibody and then immunoblotted with SUMO1 antibody (with short or long exposure). After stripping, the same membrane was detected with PTEN antibody. Quantification was analysed by ImageJ (V1.45) and the SUMO1–PTEN bands were normalized with the IgG bands. ( e ) 293T cells co-transfected with PTEN–WT or mutants K 254 R, K 266 R and K 254 R/K 266 R (KK/RR) with or without Flag-Ubc9/His-SUMO1 were lysed and treated for SUMOylation assays. Full size image PTEN activities and functions are regulated by two levels of transcriptional networks [11] , [12] , [13] and post-translational modifications, the latter including acetylation, oxidation, S-nitrosylation, phosphorylation, mono- and poly-ubiquitination. Acetylation at K 125 and K 128 mediated by PCAF (P300/CBP-associated factor) can block PTEN activity [14] . Ubiquitination at K 289 and K 13 is regulated by the E3 ubiquitin ligases NEDD4-1 [15] , [16] and WWP2 [17] ; the polyubiquitinated PTEN protein undergoes rapid degradation, whereas the monoubiquitinated form manifests the increased translocation to the nucleus. Oxidation of disulphide linkage of catalytic C 124 with C 71 mediated by reactive oxygen species also negatively regulates PTEN catalytic activity [18] . S-nitrosylation at the major site C 87 (minor sites including C 71 and C 124 ) by reactive nitrogen species inactivates its lipid phosphatase activity and mediates PTEN degradation via ubiquitination [19] . Finally, phosphorylation of PTEN mediated by a series of kinases [9] , [20] , [21] , [22] , [23] , such as RhoA-associated kinase on S 229 /T 232 and T 319 /T 321 , glycogen synthase kinase 3β on S 362 /T 366 and casein kinase 2 on S 370 /S 380 /T 382 /T 383 /S 385 , can regulate protein stability and function in cells. However, SUMOylation of PTEN has not been reported. Here we identify modification SUMO1, with SUMOylation occurring at two sites K 266 and K 254 in C2 domain of PTEN. Our data indicate that SUMO1 modification at K 266 of PTEN is essential for its tumour-suppressor function. PTEN can be SUMOylated in cells We analysed the possible SUMOylation sites of PTEN ( Supplementary Fig. S1 ) and found two consensus motifs IK 254 VE and LK 266 KD, the former located in Cβ5 and the latter located in CBR3 loop ( 263 KMLKKDK 269 ) of the C2 domain of the PTEN protein [4] ( Fig. 1a ). It has been reported that endogenous PTEN in MCF7 cells associates with Ubc9 [24] , which is a sole E2-conjugating enzyme essential for SUMOylation. We have confirmed that exogenously tagged PTEN proteins are also associated with Ubc9 in 293T cells ( Fig. 1b ). Thus, the protein interaction between PTEN and Ubc9 indicates that PTEN could be SUMOylated in cells. To verify this, we took advantage of a HeLa cell line that contains high levels of endogenous PTEN to perform in vivo SUMOylation assays [11] . As shown in Fig. 1c , affinity pulldown with Ni 2+ -NTA resin greatly enriched SUMOylated PTEN with a size of Mr ~75 kDa (the expected normal size of PTEN is 55 kDa), which is PTEN covalently conjugated with one molecule of SUMO1 (SUMO1–PTEN), in HeLa cells transfected with Flag-Ubc9/His-SUMO1, but not in cells without Flag-Ubc9/His-SUMO1. This result suggests PTEN can be SUMOylated in cells. Highly SUMOylated endogenous PTEN in SENP1 −/− MEFs Among the sentrin/SUMO-specific protease (SENP) protein family, SENP1 is the main de-SUMOylation enzyme for SUMO1-conjugated substrates [25] , [26] . We used SENP1 −/− mouse embryonic fibroblasts (MEFs) to examine the above hypothesis. Immunoblotting showed that the levels of PTEN protein were comparable in SENP1 −/− and SENP1 +/+ MEFs. Lysates were also immunoprecipitated with anti-PTEN antibody and then immunoblotted, showing that endogenous SUMO1–PTEN was detected in SENP1 −/− and SENP1 +/+ MEFs with the same size of 75 kDa by both anti-SUMO1 and anti-PTEN antibodies ( Fig. 1d ). SUMOylation of PTEN is supposed to be more easily observed in SENP1 −/− MEFs than that in SENP1 +/+ MEFs. Indeed, we observed that the SUMO1–PTEN in SENP1 −/− MEFs was four- to six-fold higher than that in SENP1 +/+ MEFs ( Fig. 1d ). These results demonstrated that endogenous PTEN can be SUMO1-modified cells. PTEN is modified by SUMO1 at both K 266 and K 254 sites To determine the SUMO acceptor sites in PTEN, mutants K 254 R, K 266 R or K 254 R/K 266 R were generated. We performed SUMOylation assays in 293T cells co-transfected wild-type (WT) PTEN, mutants K 254 R, K 266 R or K 254 R/K 266 R with or without Flag-Ubc9/His-SUMO1. As expected, one band of SUMOylated Flag-PTEN with a size of Mr ~75 kDa was observed in Ni 2+ -NTA pulldown of cells transfected with PTEN–WT plasmid ( Fig. 1e ). The double mutant K 254 R/K 266 R completely abolished SUMOylation, whereas the single mutants K 254 R or K 266 R greatly reduced SUMOylation in comparison with cells transfected with the WT construct, consistent with the notion that both K 254 and K 266 are bona fide SUMOylation sites. However, we did not observe a shift in PTEN from 55 to 95 kDa, which is presumably conjugated with two molecules of SUMO1—(SUMO1) 2 –PTEN ( Supplementary Fig. S2 ), suggesting that K 254 and K 266 are not simultaneously SUMOylated in cells. Thus, we used only two single (K 254 R and K 266 R), but not double, mutants to investigate the physiological function of SUMOylated PTEN. We have confirmed that these two point mutations do not alter other PTEN modifications, such as ubiquitination and acetylation ( Supplementary Fig. S3 ). PTEN SUMOylation suppresses anchorage-independent growth To conduct functional analyses, we generated stable PC3 luc cell lines by polyclonal lentiviral infections with Lenti-Vector, PTEN–WT, PTEN–K 254 R or PTEN–K 266 R. The expression of PTEN was comparable in all clones when assessed by western blotting ( Supplementary Fig. S4a ), indicating that these two mutations do not affect PTEN transcription rate and protein stability. Additionally, PTEN proteins, including mutants K 254 R and K 266 R, still localized predominantly to the cytoplasm ( Supplementary Fig. S4b ). To explore whether PTEN SUMOylation affects the transforming potential of each stable PC3 luc cell lines, we performed a soft agar colony-forming assay in the presence of 10% fetal bovine serum (FBS). As expected, cells transfected with PTEN–WT showed inhibition of colony growth when compared with the Lenti-Vector-transfected cells. PTEN–K 266 R-transfected cells did not suppress anchorage-independent growth, whereas PTEN–K 254 R partially lost the ability to suppress growth. Most importantly, the PTEN–K 266 R-transfected cells produced numbers and sizes of colonies equivalent to those produced by the Lenti-Vector-transfected cells ( Fig. 2a,b ). We also observed a similar pattern of results with the soft-agar colony-forming assay in the presence of 1% FBS ( Supplementary Fig. S5a ). Moreover, we generated stable 293T cells expressing PTEN–WT, PTEN–K 254 R, PTEN–K 266 R or Lenti-Vector. The colony-forming assays with these stable cell lines showed the similar pattern of results as those in stable PC3 cell lines ( Supplementary Fig. S5b ). 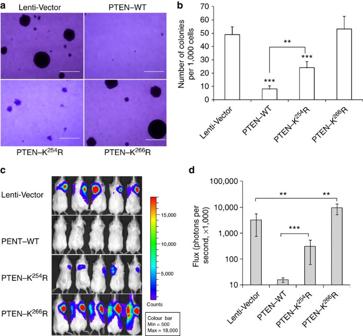Figure 2: PTEN SUMOylation is essential for its suppression of anchorage-independent growth and tumour growthin vivo. Stable PC3luctransfectants were seeded in 2 ml of medium containing 10% FBS with 0.35% agar at 1×103cells per well and layered onto the base. The photographs were taken (a), and the number of colonies was scored (b). The same scale bar (500 μm) was used in all images. Each value represents the mean±s.e.m. of three independent experiments with triplicates each. An unpaired (equal variance)t-test was performed on PTEN–WT or PTEN mutants compared with the vector control (***P<0.001), and on PTEN–WT compared with PTEN-K254R (**P<0.01). (c) Tumour growth suppression of PTEN was completely abolished by mutation of K266R. Mice were injected subcutaneously with 2.5×106PC3Luccells stably infected with Lenti-Vector, PTEN–WT, PTEN–K254R or PTEN–K266R. Tumour was assessed by bioluminescent imaging with a Xenogen IVIS imaging system at 14 days. (d) Tumour bioluminescent flux was quantified. The data is represented as the mean±s.e.m. of three independent experiments with five mice each. Differences between individual groups as indicated were analysed using thet-test (two-tailed and unpaired), andP-values of <0.01 (**) or <0.001 (***) is considered significant. Figure 2: PTEN SUMOylation is essential for its suppression of anchorage-independent growth and tumour growth in vivo . Stable PC3 luc transfectants were seeded in 2 ml of medium containing 10% FBS with 0.35% agar at 1×10 3 cells per well and layered onto the base. The photographs were taken ( a ), and the number of colonies was scored ( b ). The same scale bar (500 μm) was used in all images. Each value represents the mean±s.e.m. of three independent experiments with triplicates each. An unpaired (equal variance) t -test was performed on PTEN–WT or PTEN mutants compared with the vector control (*** P <0.001), and on PTEN–WT compared with PTEN-K 254 R (** P <0.01). ( c ) Tumour growth suppression of PTEN was completely abolished by mutation of K 266 R. Mice were injected subcutaneously with 2.5×10 6 PC3 Luc cells stably infected with Lenti-Vector, PTEN–WT, PTEN–K 254 R or PTEN–K 266 R. Tumour was assessed by bioluminescent imaging with a Xenogen IVIS imaging system at 14 days. ( d ) Tumour bioluminescent flux was quantified. The data is represented as the mean±s.e.m. of three independent experiments with five mice each. Differences between individual groups as indicated were analysed using the t -test (two-tailed and unpaired), and P -values of <0.01 (**) or <0.001 (***) is considered significant. Full size image PTEN SUMOylation suppresses tumour growth in vivo To investigate whether PTEN SUMOylation also influences tumour growth in vivo , each stable PC3 luc cell line was inoculated subcutaneously into the backs of male severe combined immunodeficiency mice. Bioluminescent imaging assessment was performed at day 14 after injection, showing that no tumours were detected in the PTEN–WT group. Tumours in the PTEN–K 254 R group grew significantly more slowly than those in both the PTEN–K 266 R and the Lenti-Vector groups, indicating that K 254 R mutation results in partial loss of the PTEN tumour suppressor activity. Notably, tumours in the PTEN–K 266 R group grew as fast as those in the Lenti-Vector group, suggesting that K 266 R mutation leads to the complete loss of PTEN tumour suppressive activity ( Fig. 2c,d ). These data suggest that K 266 SUMOylation is mainly responsible for PTEN function as a tumour suppressor. SUMO-site mutations impair PTEN downregulation of p-AKT As PTEN SUMOylation affects tumour growth in both soft agar colonies and in vivo the mouse xenograft model, we attempted to explore whether the mechanism is involved in regulation of AKT phosphorylation. Lysates from stable PC3 luc cells starved for 24 h were immunoblotted, showing that AKT phosphorylation on both T 308 and S 473 were reduced by 67–69% in PTEN–WT-transfected cells when compared with the Lenti-Vector-transfected cells. In contrast, AKT phosphorylation levels in PTEN–K 266 R-transfected cells were not significantly different from the Lenti-Vector-infected cells, whereas AKT phosphorylation was reduced by 38–39% in PTEN–K 254 R-transfected cells when compared with the Lenti-Vector-transfected cells ( Fig. 3a,b ). The patterns of phospho-AKT were the same as those of findings from both soft-agar colony-forming assay and the in vivo mouse xenograft model described above, demonstrating that K 266 SUMOylation of PTEN is required for its capability of tumour suppression through downregulation of phospho-AKT, whereas K 254 SUMOylation of PTEN is partially functional. In addition, we have also repeated these experiments in 293T cells stably expressing PTEN–WT, PTEN–K 254 R, PTEN–K 266 R or Lenti-Vector ( Supplementary Fig. S6 ), showing the results were very similar to the pattern of results obtained using stable PC3 cell lines. 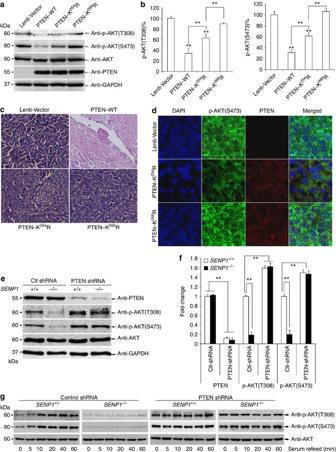Figure 3: PTEN SUMOylation is required for downregulation of AKT phosphorylation. (a) PC3luccells stably expressing WT or mutants of PTEN were starved for 24 h and lysed for immunoblotting analysis of AKT phosphorylation at Ser473and Thr308, AKT, PTEN and GAPDH. (b) Quantitation was analysed by ImageJ 1.45 (NIH, USA). The ratio of the relative intensity of p-AKT(T308) or p-AKT(S473) to total AKT is expressed. The data are presented as the mean±s.d. (n=3). Differences between individual groups as indicated were analysed using thet-test (two-tailed and unpaired), andP-values of <0.01 (**) or <0.001 (***) is considered significant. (c) Haematoxylin and eosin staining of tumour sections from the mouse xenografts at day 32 after injection of PC3luctumour cells. (d) Tumour sections were immunostained with DAPI (4′,6-diamidino-2-phenylindole (blue)) and antibodies to p-AKT(S473) (green) and PTEN (red). The same scale bar (50 μm) was used in all images. (e)SENP1−/−andSENP1+/+MEFs stably transduced by Lenti-control-shRNA or Lenti-PTEN-shRNA were starved for 24 h and lysed for immunoblotting analysis of PTEN, p-AKT(T308), p-AKT(S473), AKT and GAPDH. (f) Normalization was performed by the PTEN bands to the GAPDH bands and the p-AKT bands to the AKT bands, respectively. The data are presented as average ±s.d. (n=3). Differences between individual groups as indicated were analysed using thet-test (two-tailed and unpaired), andP-values of <0.01 (**) is considered significant. (g)SENP1−/−andSENP1+/+MEFs stably transduced by Lenti-control-shRNA or Lenti-PTEN-shRNA were serum-starved for 24 h, then treated with 10% FBS in a time course from 0 to 60 min. Lysates were immunoblotted with anti-p-AKT(T308), anti-p-AKT(S473) and anti-AKT antibodies. Figure 3: PTEN SUMOylation is required for downregulation of AKT phosphorylation. ( a ) PC3 luc cells stably expressing WT or mutants of PTEN were starved for 24 h and lysed for immunoblotting analysis of AKT phosphorylation at Ser 473 and Thr 308 , AKT, PTEN and GAPDH. ( b ) Quantitation was analysed by ImageJ 1.45 (NIH, USA). The ratio of the relative intensity of p-AKT(T 308 ) or p-AKT(S 473 ) to total AKT is expressed. The data are presented as the mean±s.d. ( n =3). Differences between individual groups as indicated were analysed using the t -test (two-tailed and unpaired), and P -values of <0.01 (**) or <0.001 (***) is considered significant. ( c ) Haematoxylin and eosin staining of tumour sections from the mouse xenografts at day 32 after injection of PC3 luc tumour cells. ( d ) Tumour sections were immunostained with DAPI (4′,6-diamidino-2-phenylindole (blue)) and antibodies to p-AKT(S 473 ) (green) and PTEN (red). The same scale bar (50 μm) was used in all images. ( e ) SENP1 −/− and SENP1 +/+ MEFs stably transduced by Lenti-control-shRNA or Lenti-PTEN-shRNA were starved for 24 h and lysed for immunoblotting analysis of PTEN, p-AKT(T 308 ), p-AKT(S 473 ), AKT and GAPDH. ( f ) Normalization was performed by the PTEN bands to the GAPDH bands and the p-AKT bands to the AKT bands, respectively. The data are presented as average ±s.d. ( n =3). Differences between individual groups as indicated were analysed using the t -test (two-tailed and unpaired), and P -values of <0.01 (**) is considered significant. ( g ) SENP1 −/− and SENP1 +/+ MEFs stably transduced by Lenti-control-shRNA or Lenti-PTEN-shRNA were serum-starved for 24 h, then treated with 10% FBS in a time course from 0 to 60 min. Lysates were immunoblotted with anti-p-AKT(T 308 ), anti-p-AKT(S 473 ) and anti-AKT antibodies. Full size image A correlation between tumour growth and AKT phosphorylation controlled by PTEN SUMOylation was observed. We stained sections from the mouse xenografts with haematoxylin and eosin, and observed that the morphology of the three xenograft tumours from the Lenti-Vector, PTEN–K 254 R and PTEN–K 266 R groups, was not different, whereas no tumour was observed in the PTEN–WT group ( Fig. 3c ). For these three xenograft tumour sections, we performed immunofluorescence analysis of PTEN and phospho-AKT. As expected, tumours in the Lenti-Vector group had no detectable endogenous PTEN protein, but high phospho-AKT. However, tumours in the PTEN–K 266 R group displayed high levels of both PTEN and phosphor-AKT, whereas tumours in the PTEN–K 254 R group showed high PTEN, but moderate phospho-AKT ( Fig. 3d ). Thus, these data provide evidence that AKT phosphorylation is relevant to tumorigenesis and controlled by PTEN SUMOylation. Endogenous SUMO1–PTEN effectively reduces phospho-AKT We asked if highly SUMOylated PTEN can more effectively reduce phospho-AKT in SENP1 −/− MEFs. Indeed, AKT phosphorylation on both T 308 and S 473 in SENP1 −/− MEFs was approximately seven-fold lower than that in SENP1 +/+ MEFs ( Supplementary Fig. S7 ). Furthermore, to verify whether PTEN is involved in downregulation of phospho-AKT in the SENP1 −/− MEFs system, SENP1 −/− and SENP1 +/+ MEFs stably transduced by Lenti-control-shRNA or Lenti-PTEN-shRNA for PTEN knockdown were serum-starved for 24 h and lysed for the analysis of phospho-AKT. As expected, AKT phosphorylation on both T 308 and S 473 in control-shRNA-transduced SENP1 −/− MEFs was much lower than those in control-shRNA-transduced SENP1 +/+ MEFs. PTEN was effectively reduced by ~90% by PTEN shRNA in both SENP1 −/− and SENP1 +/+ MEFs. Interestingly, phospho-AKT levels in both SENP1 −/− and SENP1 +/+ MEFs transduced by PTEN shRNA was almost the same and even higher than those in control-shRNA-transduced SENP1 +/+ MEFs ( Fig. 3e,f ). The MEFs were serum-starved for 24 h, then treated with 10% FBS in a time course from 0 to 60 min for analysis of phospho-AKT. The results showed that phospho-AKT was very low in control-shRNA-transduced SENP1 −/− MEFs ( Fig. 3g , the second column), whereas phospho-AKT remained high in PTEN-shRNA-transduced SENP1 +/+ ( Fig. 3g , the third column) and SENP1 −/− MEFs ( Fig. 3g , the fourth column), in the presence or absence of serum. Phospho-AKT levels were moderate at t =0 and significantly induced by serum in control-shRNA-transduced SENP1 +/+ MEFs ( Fig. 3g , the first column). These results fully support the hypothesis that SUMO1–PTEN is required for downregulation of AKT phosphorylation. SUMOylation facilitates PTEN association with the membrane To explore the underlying mechanism of SUMOylation at K 266 of PTEN that is required for the downregulation of AKT phosphorylation and consequent suppression of tumour growth, we constructed the models of PTEN and SUMO1–PTEN for molecular dynamics (MD) simulations. The simulations were based on the X-ray crystal structures of free PTEN (PDB accession code 1D5R , resolution 2.1 Å) [4] and SUMO1 (PDB accession code 2IY0 , resolution 2.7 Å) [25] . The structures of PTEN and SUMO1–PTEN (SUMO1 covalently linked to K 266 of PTEN) were taken as the starting points for MD simulations. Each MD simulation was carried out using the AMBER suite of programmes (version 8.0) with the parm99 force field (for details, see Methods). On the basis of two equilibrated dynamic trajectories, the snapshots of PTEN and SUMO1–PTEN were respectively extracted and analysed. The results revealed that PTEN in both MD systems are stable and SUMO1 modification is extended from PTEN in the system of SUMO1–PTEN during the simulation time. One eminent feature of charge topology by analysis of the NMR structure of SUMO1 is a stable bipolar surface charge, which on one side displays a positively charged surface and on the other side exhibits a large negatively charged surface [27] . More recently, it has been reported SUMO1 can bind double-stranded DNA in a sequence-independent manner through electrostatic interaction between SUMO1-positive charge surface and acidic DNA [28] . It is interesting that SUMO1–PTEN in the short MD simulation show a consensus electropositive interface contributed by K 39 , K 45 and K 46 from SUMO1, and by K 237 , K 263 and K 313 ( Fig. 4a ), indicating that SUMO1 modification of PTEN may facilitate cooperative binding of PTEN to the electronegative phospholipid membrane or its substrates by electrostatic interaction. 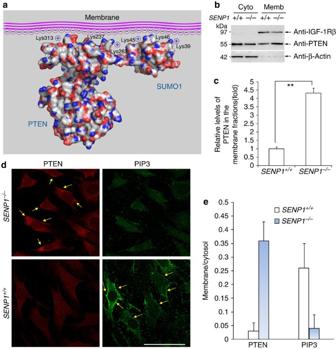Figure 4: SUMO1 modification of PTEN facilitates binding of PTEN to the phospholipid membrane. (a) MD simulations of SUMO1–PTEN binding to membrane by electrostatic interaction. (b) 10 μl per lane of each cytosolic fractions and 50 μl (usually 10 μl, but here 50 μl used for more clearly detected) of membranous protein fractions extracted fromSENP1−/−andSENP1+/+MEFs, respectively, were loaded on SDS–polyacrylamide gel electrophoresis and analysed by western blot. The anti-IGF-1Rβ as membrane marker37and anti-β-actin as cytosolic marker38were used for the loading control. (c) Quantitation was analysed by ImageJ 1.45 (NIH, USA), and normalization was performed by the PTEN bands to the IGF-1Rβ bands. The data are expressed as average ±s.d. (n=3). An unpaired (equalvariance)t-test was performed on the relative levels of PTEN in the membrane fraction ofSENP1+/+MEFs compared with those ofSENP1−/−MEFs (**P<0.01). (d) Subcellular localizations of PTEN (red) and PIP3 (green) inSENP1−/−andSENP1+/+MEFs were immunostained and monitored by confocal microscopy. The arrows represent PTEN or PIP3 plasma membrane localization. All images were identically processed and used the same scale bar (50 μm) in all images. (e) The membrane-to-cytosol ratios of PTEN and PIP3 were calculated by ImageJ. A total of 50 staining cells ofSENP1−/−orSENP1+/+MEFs, were used for quantitative analysis. Figure 4: SUMO1 modification of PTEN facilitates binding of PTEN to the phospholipid membrane. ( a ) MD simulations of SUMO1–PTEN binding to membrane by electrostatic interaction. ( b ) 10 μl per lane of each cytosolic fractions and 50 μl (usually 10 μl, but here 50 μl used for more clearly detected) of membranous protein fractions extracted from SENP1 −/− and SENP1 +/+ MEFs, respectively, were loaded on SDS–polyacrylamide gel electrophoresis and analysed by western blot. The anti-IGF-1Rβ as membrane marker [37] and anti-β-actin as cytosolic marker [38] were used for the loading control. ( c ) Quantitation was analysed by ImageJ 1.45 (NIH, USA), and normalization was performed by the PTEN bands to the IGF-1Rβ bands. The data are expressed as average ±s.d. ( n =3). An unpaired (equalvariance) t -test was performed on the relative levels of PTEN in the membrane fraction of SENP1 +/+ MEFs compared with those of SENP1 −/− MEFs (** P <0.01). ( d ) Subcellular localizations of PTEN (red) and PIP3 (green) in SENP1 −/− and SENP1 +/+ MEFs were immunostained and monitored by confocal microscopy. The arrows represent PTEN or PIP3 plasma membrane localization. All images were identically processed and used the same scale bar (50 μm) in all images. ( e ) The membrane-to-cytosol ratios of PTEN and PIP3 were calculated by ImageJ. A total of 50 staining cells of SENP1 −/− or SENP1 +/+ MEFs, were used for quantitative analysis. Full size image To confirm the above notion that SUMO1 modification of PTEN directly mediates its membrane association and consequently converting PIP3 to PIP2, we conducted a cellular fractionation assay to show that PTEN in the membrane fraction of SENP1 −/− MEFs was four-fold greater than that of SENP1 +/+ MEFs ( Fig. 4b,c ), indicating that PTEN SUMOylation is required for the recruitment of PTEN to the plasma membrane. We also showed that highly SUMOylated PTEN in SENP1 −/− MEFs intensely associated with the membrane, ablating plasma membrane PIP3 ( Fig. 4d ; Supplementary Fig. S8 ). On the contrary, low SUMOylated PTEN in SENP1 +/+ MEFs showed no membrane association, thus leading to PIP3 accumulations of the membrane ruffles. Next, we performed quantitative analysis of 50 cells for each MEFs by ImageJ software, showing that the membrane to cytosol ratios of PTEN proteins were 0.03±0.03 and 0.36±0.09 for SENP1 +/+ and SENP1 −/− MEFs, respectively. Conversely, the membrane to cytosol ratios of PIP3 were 0.26±0.07 and 0.04±0.05 for SENP1 +/+ and SENP1 −/− MEFs, respectively ( Fig. 4e ). As PIP3 is physiologically the major reaction product of PI3K, with PI(4,5)P2 being the major substrate, we used the PI3K inhibitor LY294002 to treat cells. As shown in Supplementary Fig. S9 , the immunofluorescence signal of PIP3 staining was significantly reduced, whereas immunofluorescence signal of PTEN staining was not altered in SENP1 +/+ and SENP1 −/− MEFs. These results support our MD simulation model for PTEN, in which SUMOylation facilitates binding of PTEN to the phospholipid membrane. K 266 –SUMO is mainly responsible for PTEN membrane binding As we have found that PTEN proteins are SUMOylated at K 266 and K 254 , we wanted to know which SUMOylation site is critical for the recruitment of PTEN to the plasma membrane. Thus, we performed the cellular fractionation assays with stable PC3 cell lines. As shown in Fig. 5a , PTEN was highly enriched in the plasma membrane fractions of both PTEN–WT- and PTEN–K 254 R-transfected cells, although the latter was relatively lower. Surprisingly, PTEN was not recruited to the plasma membrane of PTEN–K 266 R-transfected cells. We next used a phosphatase assay of diC 8 -PIP3 with immunoprecipitated PTEN from the same amount of above plasma membrane fractions of each stable cell line. We show that PTEN–WT-transfected cells had the highest phosphatase activity and PTEN–K 254 R mutant had an intermediate phosphatase activity, whereas the PTEN–K 266 R mutant and the Lenti-Vector-transfected cells had a basal level of activity ( Fig. 5b ). This result also accurately reflected the abundance of PTEN in those fractions. Moreover, immunofluorescence staining also confirmed that PIP3 accumulation at the plasma membrane of PTEN–K 266 R-transfected cells were also significantly increased to the similar levels as those of the Lenti-Vector-transfected cells. However, PTEN–K 254 R-transfected cells showed low levels of plasma-membrane-bound PIP3 ( Fig. 5c ). In addition, we have also repeated the cellular fractionation and phosphatase assays in 293T cells transiently transfected with the empty vector, PTEN–WT, PTEN–K 254 R or PTEN–K 266 R plasmids, together with SUMO1 and Ubc9, and showed comparable results ( Fig. 5d,e ) to those of stable PC3 cell lines. Taken together, the above results correlated well with the tumour suppressor phenotype, including mouse xenograft and soft agar colony, and demonstrated that SUMOylation at K 266 is mainly responsible for the recruitment of PTEN to the plasma membrane. 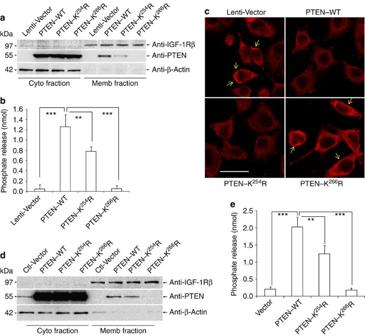Figure 5: SUMOylation at K266but not K254is responsible for the recruitment of PTEN to the plasma membrane. (a) A volume of 10 μl per lane of each cytosolic fraction and membranous protein fraction extracted from PC3luccells stably expressing WT or mutants of PTEN, respectively, was loaded on SDS–polyacrylamide gel electrophoresis and western blotted with anti-PTEN, anti-IGF-1Rβ and anti-β-actin antibodies. (b) Malachite green phosphatase assay using proteins immunoprecipitated with anti-PTEN antibody from equal amounts of membranous fraction extracted from 1×108of each stable PC3luccell line expressing WT or mutants of PTEN. The data are presented as average ±s.d. (n=4). Differences between individual groups as indicated were analysed using thet-test (two-tailed and unpaired), andP-values of <0.01 (**) or <0.001 (***) is considered significant. (c) PC3luccells stably expressing WT or mutants of PTEN were immunostained with anti-PIP3 antibody and monitored by confocal microscopy. The arrows represent PIP3 plasma membrane localization. All images were identically processed and the same scale bar (25 μm) was used in all images. (d) A volume of 10 μl per lane of each cytosolic fraction and membranous protein fraction extracted from 293T cells transiently transfected with the empty vector, Flag-PTEN–WT, –K254R or –K266R together with or without HA-Ubc9 and His-SUMO1, respectively, was loaded on SDS–polyacrylamide gel electrophoresis and western blotted with anti-PTEN, anti-IGF-1Rβ and anti-β-actin antibodies. (e) Malachite green phosphatase assay using proteins immunoprecipitated with anti-PTEN antibody from equal amounts of membranous fraction extracted from 3×107of each 293T cells transiently transfected with the empty vector, Flag-PTEN–WT, –K254R or –K266R together with or without HA-Ubc9 and His-SUMO1. The data are presented as average ±s.d. (n=4). Differences between individual groups as indicated were analysed using thet-test (two-tailed and unpaired), andP-values of <0.01 (**) or <0.001 (***) is considered significant. Figure 5: SUMOylation at K 266 but not K 254 is responsible for the recruitment of PTEN to the plasma membrane. ( a ) A volume of 10 μl per lane of each cytosolic fraction and membranous protein fraction extracted from PC3 luc cells stably expressing WT or mutants of PTEN, respectively, was loaded on SDS–polyacrylamide gel electrophoresis and western blotted with anti-PTEN, anti-IGF-1Rβ and anti-β-actin antibodies. ( b ) Malachite green phosphatase assay using proteins immunoprecipitated with anti-PTEN antibody from equal amounts of membranous fraction extracted from 1×10 8 of each stable PC3 luc cell line expressing WT or mutants of PTEN. The data are presented as average ±s.d. ( n =4). Differences between individual groups as indicated were analysed using the t -test (two-tailed and unpaired), and P -values of <0.01 (**) or <0.001 (***) is considered significant. ( c ) PC3 luc cells stably expressing WT or mutants of PTEN were immunostained with anti-PIP3 antibody and monitored by confocal microscopy. The arrows represent PIP3 plasma membrane localization. All images were identically processed and the same scale bar (25 μm) was used in all images. ( d ) A volume of 10 μl per lane of each cytosolic fraction and membranous protein fraction extracted from 293T cells transiently transfected with the empty vector, Flag-PTEN–WT, –K 254 R or –K 266 R together with or without HA-Ubc9 and His-SUMO1, respectively, was loaded on SDS–polyacrylamide gel electrophoresis and western blotted with anti-PTEN, anti-IGF-1Rβ and anti-β-actin antibodies. ( e ) Malachite green phosphatase assay using proteins immunoprecipitated with anti-PTEN antibody from equal amounts of membranous fraction extracted from 3×10 7 of each 293T cells transiently transfected with the empty vector, Flag-PTEN–WT, –K 254 R or –K 266 R together with or without HA-Ubc9 and His-SUMO1. The data are presented as average ±s.d. ( n =4). Differences between individual groups as indicated were analysed using the t -test (two-tailed and unpaired), and P -values of <0.01 (**) or <0.001 (***) is considered significant. Full size image PTEN-controlled tumorigenesis is dependent on K 266 –SUMO To investigate the structural basis of the CBR3 loop in PTEN-controlled tumorigenesis, MD simulations, and structural and functional analysis were performed on PTEN and its four mutants. The results show that the conformation of the CBR3 loop could significantly change, owing to sequential multiple replacements of PTEN M-CBR3 (PTEN 263 AAGAADA 269 ) [4] . The most greatest deviation of the loop in PTEN 263 AAGAADA 269 is around residue 266 and the positively charged property of the loop has been eliminated, which could lead to a lower ability to bind the membrane [4] . On the contrary, single mutations at residue 266 had little effect on the perturbation of the CBR3 loop and the whole PTEN conformation (the root-mean-square deviation for the Cα atoms <1.8 Å) in the solvents. These mutations ranged from a similar positively charged residue (PTEN–K 266 R) to a polar residue (PTEN–K 266 Q), to a non-polar residue (PTEN–K 266 A), in comparison with WT PTEN ( Fig. 6a ). Although the simulation times were limited, the conserved conformations in the PTEN–K 266 mutants provide a clue that these various mutants could have the same biological contribution. To verify this, we also generated PC3 cell lines stably expressing PTEN–K 266 Q, PTEN–K 266 A or PTEN–G 129 R, and conducted the soft-agar anchorage-independent growth assays with these mutants. Three point mutants K 266 R, K 266 Q or K 266 A produced soft-agar colonies equivalent in size and number to those produced by the Lenti-Vector- and PTEN–G 129 R-transfected cells (as a positive control) [29] ( Fig. 6b,c ). Furthermore, we determined the levels of phospho-AKT, showing that PTEN–WT effectively inhibited AKT phosphorylation on both T 308 and S 473 , whereas all other mutants including K 266 R, K 266 Q, K 266 A and PTEN–G 129 R completely lost this ability ( Fig. 6d ). Therefore, the tumour formation of PTEN–K 266 mutants is ascribed to SUMOylation deficiency instead of a conformational change. 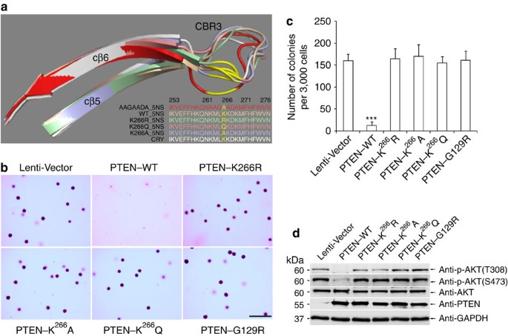Figure 6: PTEN-controlled tumorigenesis is K266-SUMO-dependent and not due to changes in PTEN conformation. (a) Superimposition of the CBR3 loops isolated from the structures of PTEN and PTEN mutants in both crystal and MD simulations. The sequence alignment of cβ5-CBR3-cβ6 (defined by Leeet al.)4from the structures is shown in the lower right corner. Residue K266is highlighted in yellow in both sequences and structures. AAGAADA_5NS (PTEN263AAGAADA269at 5-ns MD simulation); WT_5NS (WT PTEN at 5-ns MD simulation); K266R_5NS (PTEN K266R at 5-ns MD simulation); K266Q_5NS (PTEN K266Q at 5-ns MD simulation); K266A_5NS (PTEN K266A at 5-ns MD simulation); CRY (PTEN crystal 1D5R). (b) Stable PC3luccells stably expressing WT PTEN or mutants (including K266R, K266A, K266Q and G129R) were seeded in 2 ml of medium containing 10% FBS with 0.35% agar at 3×103cells/ per well and layered onto the base. The photographs of the cells growing in plate and of the colonies developed in soft agar were taken 2 weeks after seeding. All images were identically processed and the same scale bar (500 μm) was used in all images. (c) The number of colonies was scored. Each value represents the mean±s.e.m. of three independent experiments with triplicates each. An unpaired (equalvariance)t-test was performed on Lenti-Vector or PTEN mutants compared with PTEN–WT (***,P<0.001). (d) PC3luccells stably expressing WT PTEN and mutants were starved for 24 h, and then lysed for immunoblotting analysis of AKT phosphorylation at Ser473and Thr308, AKT, PTEN and GAPDH. Figure 6: PTEN-controlled tumorigenesis is K 266 -SUMO-dependent and not due to changes in PTEN conformation. ( a ) Superimposition of the CBR3 loops isolated from the structures of PTEN and PTEN mutants in both crystal and MD simulations. The sequence alignment of cβ5-CBR3-cβ6 (defined by Lee et al .) [4] from the structures is shown in the lower right corner. Residue K 266 is highlighted in yellow in both sequences and structures. AAGAADA_5NS (PTEN 263 AAGAADA 269 at 5-ns MD simulation); WT_5NS (WT PTEN at 5-ns MD simulation); K 266 R_5NS (PTEN K 266 R at 5-ns MD simulation); K 266 Q_5NS (PTEN K 266 Q at 5-ns MD simulation); K 266 A_5NS (PTEN K 266 A at 5-ns MD simulation); CRY (PTEN crystal 1D5R). ( b ) Stable PC3 luc cells stably expressing WT PTEN or mutants (including K 266 R, K 266 A, K 266 Q and G 129 R) were seeded in 2 ml of medium containing 10% FBS with 0.35% agar at 3×10 3 cells/ per well and layered onto the base. The photographs of the cells growing in plate and of the colonies developed in soft agar were taken 2 weeks after seeding. All images were identically processed and the same scale bar (500 μm) was used in all images. ( c ) The number of colonies was scored. Each value represents the mean±s.e.m. of three independent experiments with triplicates each. An unpaired (equalvariance) t -test was performed on Lenti-Vector or PTEN mutants compared with PTEN–WT (***, P <0.001). ( d ) PC3 luc cells stably expressing WT PTEN and mutants were starved for 24 h, and then lysed for immunoblotting analysis of AKT phosphorylation at Ser 473 and Thr 308 , AKT, PTEN and GAPDH. Full size image Furthermore, to more strongly support the hypothesis that the mutation of K 266 inhibits PTEN SUMOylation-dependent membrane recruitment, but does not alter the conformation of PTEN thereby hindering its recruitment to the plasma membrane, we made Flag-tagged SUMO1–PTEN (WT, K 254 R or K 266 R) fusion expression constructs and generated stable PC3 cell lines by lentiviral infections with these new constructs ( Fig. 7a ). We conducted western blotting analysis of phospho-AKT ( Fig. 7b ), the soft-agar colony-forming assays ( Fig. 7c ) and cellular fraction assays ( Fig. 7d ). Indeed, all these artificially SUMOylated forms of PTEN were equally recruited to the membrane, although relatively less so when compared with PTEN in the cytoplasmic fractions, which is probably due to the fast dynamic association between PTEN and the inner face of plasma membrane. As expected, similar to PTEN–WT– sumo1 , both PTEN–K254R– sumo1 and PTEN–K266R– sumo1 reversed the phenotypic observations of inhibition of phospho-AKT ( Fig. 7b ) and anchorage-independent growth ( Fig. 7c ). These results demonstrate that PTEN SUMOylation in PTEN-null PC3 cells is indeed important for PTEN membrane recruitment. 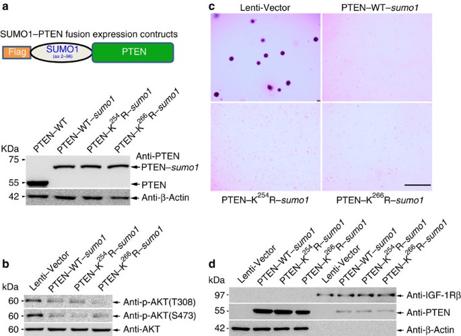Figure 7: SUMOylated forms of PTEN by gene fusion are recruited to the plasma membrane and reverse the phenotypic observations. (a) SUMO1–PTEN fusion expression constructs Lenti-PTEN–WT–sumo1, PTEN–K254R–sumo1and PTEN–K266R–sumo1were generated (detail seeSupplementary Methods) and their structure is shown. PC3luccells were infected with the prepared pseudovirus containing the lentivirus expression constructs Lenti-PTEN–WT or above SUMO1–PTEN fusion expression constructs. Stably transduced cells selected by puromycin were lysed and immunoblotted with anti-PTEN and anti-β-actin antibodies. Three of SUMO1–PTEN fusion proteins were expressed comparable to the same size of Mr ~70 kDa, whereas the PTEN–WT without fusion of SUMO1 was expressed with a normal size of Mr ~55 kDa. (b) Point mutations of K266R and K254R that impair PTEN function in downregulation of AKT phosphorylation were phenotypically rescued by covalent attachment of SUMO1 to PTEN by gene fusion. PC3luccells stably expressing Lenti-PTEN–WT–sumo1, PTEN–K254R–sumo1and PTEN–K266R–sumo1were starved for 24 h, and then lysed for immunoblotting analysis of AKT phosphorylation at Ser473and Thr308. (c) The effect of SUMO1–PTEN fusion proteins on anchorage-independent growth was assessed using a soft agar colony assay. PC3luccells stably expressing Lenti-PTEN–WT–sumo1, PTEN–K254R–sumo1and PTEN–K266R–sumo1(including control PC3luccells with Lenti-Vector) were seeded in 2 ml of medium containing 10% FBS with 0.35% agar at 3×103cells per well and layered onto the base. The photographs of the cells growing in plate and of the colonies developed in soft agar were taken 2 weeks after seeding. All images were identically processed and the same scale bar (500 μm) was used in all images. (d) A volume of 10 μl per lane of each cytosolic fraction and membranous protein fraction extracted from PC3luccells stably expressing Lenti-Vector, PTEN–WT–sumo1, PTEN–K254R–sumo1and PTEN–K266R–sumo1, respectively, was loaded on SDS–polyacrylamide gel electrophoresis and western blotted with anti-PTEN, anti-IGF-1Rβ and anti-β-actin antibodies. Figure 7: SUMOylated forms of PTEN by gene fusion are recruited to the plasma membrane and reverse the phenotypic observations. ( a ) SUMO1–PTEN fusion expression constructs Lenti-PTEN–WT– sumo1 , PTEN–K 254 R– sumo1 and PTEN–K 266 R– sumo1 were generated (detail see Supplementary Methods ) and their structure is shown. PC3 luc cells were infected with the prepared pseudovirus containing the lentivirus expression constructs Lenti-PTEN–WT or above SUMO1–PTEN fusion expression constructs. Stably transduced cells selected by puromycin were lysed and immunoblotted with anti-PTEN and anti-β-actin antibodies. Three of SUMO1–PTEN fusion proteins were expressed comparable to the same size of Mr ~70 kDa, whereas the PTEN–WT without fusion of SUMO1 was expressed with a normal size of Mr ~55 kDa. ( b ) Point mutations of K 266 R and K 254 R that impair PTEN function in downregulation of AKT phosphorylation were phenotypically rescued by covalent attachment of SUMO1 to PTEN by gene fusion. PC3 luc cells stably expressing Lenti-PTEN–WT– sumo1 , PTEN–K 254 R– sumo1 and PTEN–K 266 R– sumo1 were starved for 24 h, and then lysed for immunoblotting analysis of AKT phosphorylation at Ser 473 and Thr 308 . ( c ) The effect of SUMO1–PTEN fusion proteins on anchorage-independent growth was assessed using a soft agar colony assay. PC3 luc cells stably expressing Lenti-PTEN–WT– sumo1 , PTEN–K 254 R– sumo1 and PTEN–K 266 R– sumo1 (including control PC3 luc cells with Lenti-Vector) were seeded in 2 ml of medium containing 10% FBS with 0.35% agar at 3×10 3 cells per well and layered onto the base. The photographs of the cells growing in plate and of the colonies developed in soft agar were taken 2 weeks after seeding. All images were identically processed and the same scale bar (500 μm) was used in all images. ( d ) A volume of 10 μl per lane of each cytosolic fraction and membranous protein fraction extracted from PC3 luc cells stably expressing Lenti-Vector, PTEN–WT– sumo1 , PTEN–K 254 R– sumo1 and PTEN–K 266 R– sumo1 , respectively, was loaded on SDS–polyacrylamide gel electrophoresis and western blotted with anti-PTEN, anti-IGF-1Rβ and anti-β-actin antibodies. Full size image Recent studies have revealed that the presence of SUMOylated proteins occurs not only in the nucleus, but also in other cellular compartments, including the cytoplasm, mitochondria, endoplasmic reticulum and the plasma membrane [30] . PTEN is mainly found in the cytoplasm as a lipid phosphatase that dephosphorylates its substrate at the plasma membrane, but is also found in the nucleus [15] , [16] . In this study, we have confirmed that PTEN can be modified by SUMO1 in HeLa cells ( Fig. 1c ), 293T cells ( Fig. 1e ) and PC3 cells ( Supplementary Fig. S2 ) using His-tagged SUMO1 conjugates bound to Ni 2+ -NTA beads. Importantly, we used immunoprecipitation and western blotting to show the high level of endogenous SUMOylated PTEN in SENP1 −/− MEFs ( Fig. 1d ). In fact, PTEN has also been found to directly translocate to the plasma membrane in certain cell lines and under specific conditions [3] , [20] , [31] . Our finding that SUMO1 modification of PTEN increases PTEN binding to the plasma membrane ( Figs 4 , 5 and 7 ) may explain why a small fraction of PTEN acts through the dynamic interaction with the inner face of plasma membrane [2] . Most SUMO targets appear to be SUMOylated to a small percentage at steady state; nevertheless, this low-level SUMOylation causes large effects [30] . Dynamic cycles of SUMOylation and de-SUMOylation transiently occur within seconds [32] , and PTEN binds to the plasma membrane for a few hundred milliseconds, which is sufficient to dephosphorylate PIP3 [2] . Thus, in view of these time frames, it is reasonable to assume that PTEN SUMOylation and PTEN membrane association can occur in this time. As previous studies have shown [4] , [5] , [6] , PTEN binds to phospholipid membranes via its C2 domain, in which the CBR3 loop has a central role in the binding. The solvent-exposed loop has four positively charged lysines (K 263 , K 266 , K 267 and K 269 ) and two hydrophobic residues (M 264 and L 265 ). A mutant of this region, PTEN M-CBR3 ( 263 AAGAADA 269 ) [4] , shows reduced affinity for membranes in vitro compared with WT PTEN. In this study, we found K 266 in the CBR3 loop is SUMO modified, and the K 266 mutant has been revealed to contribute to increased tumour formation ( Fig. 2c ). To predict the structural and functional relationship of K 266 , the MD simulations on PTEN-WT and its mutants, including K 266 R, K 266 A and K 266 Q, were performed and the results showed that the conformations in the PTEN K 266 mutants are conserved in 5-ns trajectories ( Fig. 6a ). Considering the temporal and spatial features of PTEN function, long simulation of PTEN systems in the presence of a negatively charged bilayer can provide more convincing evidences in the mechanism studies of both CBR3 SUMOylation and membrane recruitment. Nevertheless, a series of very short MD simulations in this study have been employed to simply predict potential effects of PTEN mutants; these need to be verified with further biological experiments. However, these various mutants with the same biological contribution have been validated by the soft agar anchorage-independent growth assays ( Fig. 6b,c ) and the determination of phospho-AKT levels ( Fig. 6d ). Therefore, PTEN-controlled tumorigenesis is more likely to be K 266 –SUMO-dependent, but not due to changes in PTEN conformation. It has been proposed in the PTEN open/closed model that phosphorylation at S 370 /S 380 /T 382 /T 383 /S 385 of the C-terminal tail regulate membrane association [3] , [33] . This model is also involved in binding of the C2 domain to phosphatidylserine [4] and the PIP2-binding motif to PIP2 [7] , [34] . We have provided evidence that a consensus electropositive interface in SUMO1–PTEN facilitates cooperative binding of PTEN with the electronegative phospholipid membrane or its substrates by electrostatic interaction. Phosphorylation leads to a closed conformation that prevents PTEN association with the plasma membrane [9] , [10] ; however, if taken into account the electrostatic status, phosphorylation actually supplies negative charges. Therefore, SUMOylation appears to be a positive regulator in controlling PTEN membrane association, whereas phosphorylation is a negative regulator that may neutralize SUMOylation through intramolecular electrostatic interactions. This hypothesis remains to be validated in the future. We detected enhanced tumour proliferation when K 254 was mutated, but this was less than the K 266 mutant, which elicits the same tumorigenic phenotype as seen in the PTEN-null condition ( Fig. 2 ). From this observation, it seems that both K 266 and K 254 are important in regulating tumour formation, but more so when K 266 is mutated. According to the principle of electrostatic interaction, the SUMOylation of either K 254 or K 266 could provide charge to help PTEN in the process of membrane binding. However, K 254 is located in the rigid β-strand of the Cβ5 domain and K 266 is located in the flexible CBR3 loop; thus, K 266 has more potential for conformational changes to induce biological function. This is in agreement with previous studies that the CBR3 loop is necessary for membrane binding. In addition, the SUMO1 protein contains more than 90 residues, and the requirement of space near the modified site is much larger than for other posttranslational modifications (for example, methylation, acetylation, phosphorylation), leading to an unfavourable factor for single SUMOylation of K 254 embedded in the Cβ5 domain or dual SUMOylation of adjacent K 254 and K 266 . In summary, as shown in Fig. 8 , our data unravel an unexpected regulatory mechanism that PTEN SUMOylation is required for inhibition of the PTEN/PI3K/AKT pathway. SUMO1 modification of PTEN at K 266 mainly facilitates cooperative binding of PTEN to the electronegative phospholipid membrane by electrostatic interaction, then dephosphorylating PIP3 to PIP2, consequently blocking AKT activation and suppressing anchorage-independent cell proliferation and tumour growth in vivo . Our findings might also have important implications in cancer aetiology and cancer therapy, as dysregulation of the PTEN/PI3K/AKT pathway is associated with diverse cancers. 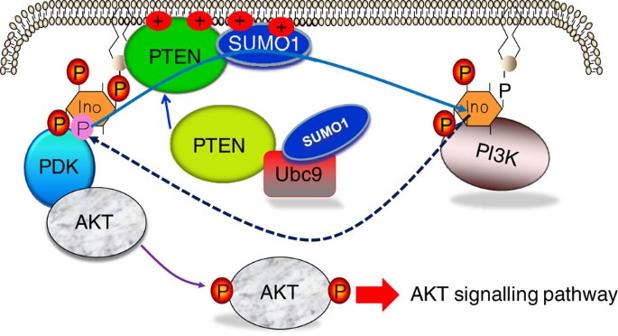Figure 8: A novel regulatory mechanism for the PTEN–PI3K–AKT pathway. A receptor tyrosine kinase (RTK) activated by its ligand phosphorylates PI3K to convert PIP2 to PIP3. PIP3 serves as a second messenger and together with PDKs activates AKT. Activated AKT, by phosphorylation, mediates the activation and inhibition of several targets, resulting in cell growth, proliferation, survival and transformation. On the other hand, the tumour suppressor PTEN as a lipid phosphatase antagonizes PI3K function and consequently inhibits downstream signalling through Akt. SUMO1 modification at K266of PTEN mainly facilitates cooperative binding of PTEN to the electronegative phospholipid membrane by electrostatic interaction, then dephosphorylating PIP3 to PIP2, consequently blocking AKT activation and suppressing anchorage-independent cell proliferation and tumour growthin vivo. Figure 8: A novel regulatory mechanism for the PTEN–PI3K–AKT pathway. A receptor tyrosine kinase (RTK) activated by its ligand phosphorylates PI3K to convert PIP2 to PIP3. PIP3 serves as a second messenger and together with PDKs activates AKT. Activated AKT, by phosphorylation, mediates the activation and inhibition of several targets, resulting in cell growth, proliferation, survival and transformation. On the other hand, the tumour suppressor PTEN as a lipid phosphatase antagonizes PI3K function and consequently inhibits downstream signalling through Akt. SUMO1 modification at K 266 of PTEN mainly facilitates cooperative binding of PTEN to the electronegative phospholipid membrane by electrostatic interaction, then dephosphorylating PIP3 to PIP2, consequently blocking AKT activation and suppressing anchorage-independent cell proliferation and tumour growth in vivo . Full size image Cell cultures Human embryonic kidney 293T, 293FT and HeLa cells were cultured in Dulbecco's modified Eagle's medium (DMEM) containing 10% fetal calf serum (FCS; Hyclone), penicillin and streptomycin (Invitrogen) at 37 °C and 5% CO 2 . PC3 luc expressing a firefly luciferase can be used for living imaging [35] . PC3 luc cells were cultured in RPMI1640 in 10% FCS, penicillin and streptomycin at 37 °C and 5% CO 2 . MEF cells from SENP1 homozygous null ( SENP1 −/− ) and WT ( SENP1 +/+ ) mice [36] , which was provided by Dr J. K. Cheng in SJTU-SM, were cultured in DMEM with 10% FBS. SENP1 +/+ and SENP1 −/− MEFs were generated and maintained according to the protocol of Cheng et al . [36] Cell transfection was performed using Lipofectamine 2000 (Invitrogen). Soft agar colony assay The effect of PTEN and its mutants on anchorage-independent growth was assessed using a soft agar colony assay. Briefly, this assay was performed in six-well plates with a base of 2 ml of medium containing 10 or 1% FBS with 0.6% Bacto agar (Amresco). Stable PC3 luc transfectants were seeded in 2 ml of medium containing 10 or 1% FBS with 0.35% agar at 1×10 3 or 1×10 4 cells per well and layered onto the base, respectively. The photographs of the cells growing in the plate and of the colonies developed in soft agar were taken, and the number of colonies was scored by ImageJ V1.45 (NIH, USA). Analysis of SUMO1-modified protein SUMO1 modification of PTEN was analysed in 293T, HeLa or PC3 cells by the method of His-tagged SUMO1 conjugates binding to Ni 2+ -NTA beads as previously described [11] . For analysis of endogenous SUMO1–PTEN, SENP1 −/− and SENP1 +/+ MEFs were lysed in NEM-RIPA buffer, and 1500 μg of lysates were used for immunoprecipitation with 5 μl of anti-PTEN (26H9) antibody, then immunoblotted with anti-SUMO1 and anti-PTEN antibodies (dilution 1:1000). Extraction of membrane/cytosol fractions A total of 8−10×10 6 cells were used for each extraction, and the extractions were performed according to the manufacturer's instructions of FractionPREP Cell Fractionation kit (BioVision, CA, USA). Both subcellular fractions were further resuspended in 400 μl of buffer, and usually 10 μl per lane of each cytosolic and membranous protein fractions were loaded on SDS–polyacrylamide gel electrophoresis and western blotted. The anti-IGFIRβ as a membrane marker [37] and anti-β-actin as a cytosolic marker [38] were used for the loading control. Phosphatase assays Equal amounts of membranous fractions from 1×10 8 of each stable PC3 luc cell line expressing WT PTEN or mutants were used for immunoprecipitation with 5 μl of anti-PTEN (26H9; Fig. 5b ). Equal amounts of membranous fractions from 3×10 7 of each 293T transiently transfected with the empty vector, Flag-PTEN–WT, –K 254 R or –K 266 R, together with or without HA-Ubc9 and His-SUMO1, were used for immunoprecipitation with 5 μl of anti-Flag antibody ( Fig. 5e ). According to the manufacturer's protocol of Malachite Green Phosphatase Assay Kit (Echelon, Salt Lake City, Utah), the phosphatase reactions with water-soluble diC8-PIP3 (Echelon) were performed with the above immunoprecipitated proteins. Mouse xenograft models Murine xenografts were established in 6- to 8-week-old male severe combined immunodeficiency mice using PC3 luc cells, which were stably infected with Lenti-Vector, PTEN–WT, PTEN–K 254 R and PTEN–K 266 R, respectively. Per injection site, a total volume of 100 μl containing 2.5×10 6 PC3 luc cells were inoculated subcutaneously into the backs. Tumour volume was assessed by imaging isofluorane-anaesthetized mice with the IVIS system (Xenogen, Alameda, CA). Images were obtained 10 min after intraperitoneal injection of 1.5 mg (approx. 75 mg kg −1 ) D-luciferin (Xenogen) in 100 μl of PBS. The light emitted by luciferase-expressing tumours was quantified using Living Image Version 2.50 (Wavemetrics, Lake Oswego, OR). A heatmap image corresponding to photons/second/cm 2 /steradian (blue lowest and red highest) was superimposed over the reflected light image of the animals for tumour localization. A rectangular region of interest encompassing the mouse head and body was replicated between images, images were adjusted to identical luminescent scales, and bioluminescence reported as total flux for the region in photons per second. Animals were imaged on day 14 and 21. The data is represented as the mean±s.e.m. of three independent experiments with five mice each. In vivo bioluminescent numerical data accounting for tumour growth was compared between groups using one-way repeated-measures analysis of variance for significance of intergroup comparisons. Statistical analysis was performed using Prism 5 (GraphPad Software, La Jolla, CA). All animal studies were conducted with the approval and guidance of Shanghai Jiao Tong University Medical Animal Ethics Committees. Immunofluorescene and confocal microscopy Immunofluorescene staining method was performed as previously described [11] . Briefly, SENP1 −/− and SENP1 +/+ MEFs were directly seeded into the uncoated 35-mm dishes at a density of 1.0×10 5 cells. After 24 h, cells were treated with LY294002 (20 μM) or vehicle (DMSO) for 30 min, then washed in PBS once, fixed with 4% freshly prepared formaldehyde in PBS for 8–10 min, and then washed three times with PBS. Cells were permeabilized with 0.1% Saponin (or Triton 100)/PBS for 15 min, blocked in 2.5% normal goat serum in 0.1% Saponin (or Triton 100)/PBS for 30 min–24 h, incubated in the primary antibodies anti-PTEN(138G6, rabbit monoclonal immunoglobulin G, dilution 1:50) and anti-PI(3,4,5)P 3 (Z-P345b, mouse monoclonal immunoglobulin G, dilution 1:50) diluted in blocking solution for 1 h, washed three times with blocking solution and then incubated in the second antibody (Alexa 568 anti rabbit, or Alexa 488 anti mouse, dilution 1:500) in blocking solution for 30 min. The cells were then washed twice with blocking solution, and once with PBS. DAPI (4′,6-diamidino-2-phenylindole) was added for DNA staining. Images were taken with a Zeiss LSM710 Confocal Microscope (Carl Zeiss, Jena, Germany). All confocal images were analysed and quantified using ImageJ v. 1.45 ( http://rsb.info.nih.gov/ij / ). The membrane-to-cytosol ratio of respective experiments was calculated on single Z- planes using the methods developed by Janetopoulos et al . [39] and Ulrich et al . [40] For each of MEFs, 50 staining cells were used for quantitative analysis and statistical analysis ( Fig. 4d ). Molecular models of PTEN and SUMOylated PTEN The models of PTEN, SUMOylated PTEN (SUMO1–PTEN) and four mutated PTEN (K 266 R, K 266 Q, K 266 A, M-CBR3-- 263 AAGAADA 269 ) for the MD simulations were constructed based on the X-ray crystal structures of free PTEN (1D5R, resolution 2.1 Å) [4] and SUMO1 (2IY0, resolution 2.7 Å) [25] . The side chains with missing coordinates were reconstructed using the fragment library of the Biopolymer module in Sybyl version 6.8 (Tripos, St Louis, MO). The modified structures were subjected to energy minimization in Sybyl6.8, using the steepest descent method up to the gradient tolerance of 0.05 kcal per mol·Å to relieve possible steric clashes and overlaps of side chains. The three-dimensional structural model of SUMO1–PTEN was built up using the xLeap module in the AMBER suite (version 8.0). MD simulations The structures of six models were taken as the starting points for MD simulations. We performed the MD simulation of PTEN–SUMO1 after modelling, to relax the conformation of PTEN–SUMO1 in solution and remove unfavourable contacts arising from the initial rigid-body modelling, whereas other MD simulations on PTEN mutants were used to investigate the structural basis and conformational changes of the CBR3 loop. Each MD simulation was carried out using the AMBER suite of programmes (version 8.0) with the parm99 force field [41] . Each structure was prepared by using the xLeap module in AMBER, in which protons were added to the structure. All ionizable side chains were maintained in their standard protonation states at pH 7.0. The proteins were solvated in cubic box of water molecules, with a water thickness extending at least 10 Å apart from the protein surface. To avoid the instability that might occur during the MD simulations, the solvated system was subjected to minimization for 5000 cycles with protein restrained and followed by another 5,000 cycles with the whole system relaxed. Then, the system was gradually heated from 0 to 300 K during the first 60 ps by three intervals, followed by equilibrium for 80 ps under constant volume and temperature condition. Afterwards, the system was switched to constant pressure and temperature condition and equilibrated for 100 ps to adjust the system to a correct density. Finally, the production simulations were carried out in the absence of any restraint under constant pressure and temperature condition and two 5-ns MD simulations were then conducted on the PTEN and SUMO1–PTEN to probe the function of SUMOylation. This protocol was applied to all of the simulation systems. All the MD simulations were performed using the parallel version of PMEMD in AMBER suit. The particle mesh Ewald method was employed to calculate the long-range electrostatic interactions, whereas the lengths of the bonds involving hydrogen atoms were fixed with the SHAKE algorithm [42] . During the simulations, the integration time step of 2 fs was adopted and structural snapshots were flushed every 500 steps (1 ps). The non-bonded cutoff was set to 10.0 Å, and the non-bonded pair list was updated every 25 steps. Each production simulation was coupled to a 300 K thermal bath at 1.0 atmospheric pressure by applying the Berendsen algorithm. The temperature and pressure coupling constants were set to 2.0 and 1.0 ps, respectively. How to cite this article: Huang, J. et al . SUMO1 modification of PTEN regulates tumorigenesis by controlling its association with the plasma membrane. Nat. Commun. 3:911 doi: 10.1038/ncomms1919 (2012).